PH13improves soybean shade traits and enhances yield for high-density planting at high latitudes Shading in combination with extended photoperiods can cause exaggerated stem elongation (ESE) in soybean, leading to lodging and reduced yields when planted at high-density in high-latitude regions. However, the genetic basis of plant height in adaptation to these regions remains unclear. Here, through a genome-wide association study, we identify a plant height regulating gene on chromosome 13 ( PH13 ) encoding a WD40 protein with three main haplotypes in natural populations. We find that an insertion of a Ty1/Copia -like retrotransposon in the haplotype 3 leads to a truncated PH13 H3 with reduced interaction with GmCOP1s, resulting in accumulation of STF1/2, and reduced plant height. In addition, PH13 H3 allele has been strongly selected for genetic improvement at high latitudes. Deletion of both PH13 and its paralogue PHP can prevent shade-induced ESE and allow high-density planting. This study provides insights into the mechanism of shade-resistance and offers potential solutions for breeding high-yielding soybean cultivar for high-latitude regions. Soybean ( Glycine max (L.) Merr.) is an economically important crop, accounting for 59% of the oilseed production and providing 70% of the plant protein for human and animal consumption worldwide (SoyStats, 2023) [1] . To meet the demands of an ever-growing population and to continuously improve the living standards, it is estimated that the global soybean yield must be doubled by 2050 [2] , [3] . Soybean is a short-day plant (SDP) that originated in the temperate regions of China (between 32 and 40°N) [4] . However, traditional soybean varieties are restricted to narrow range of latitudes due to their high photoperiod sensitivity, resulting in traits such as maturity time and plant architecture being affected [5] , [6] . The introduction of new genetic resources has enabled the expansion of cultivation worldwide. In particular, the long juvenile trait (LJ) has been successfully utilized since the 1970s for the breeding of cultivars suitable for lower latitudes (below 22°), making Brazil the largest producer of soybean in the world [7] , [8] , [9] . High latitudes are also essential areas for soybean production. In 2021, China’s three northeastern provinces (Heilongjiang, Jilin, and Liaoning at latitudes of over 40°N) accounted for 48.71% of the country’s total soybean production (NBSC, 2022). However, the worldwide cultivation of soybean at high latitudes (over 40°N) only produced less than 20% of the total yield, suggesting a great potential to boost global yield by cultivation of soybean in these regions including the far Russia East, Canada, the Northern United States, and the Northeast of China. High latitudes have long-day photoperiods which can induce an extended maturity period and excessive stem growth, impeding the adaptation of soybean varieties to their short frost-free farm seasons. Several flowering time genes, including the early flowering locus ( E1 - E4 ) [10] , [11] , [12] , [13] , Tof5 [14] , two homologs of PSEUDO-RESPONSE-REGULATOR3 , Tof11 and Tof12 [15] , [16] , [17] , have been reported to be utilized for breeding of soybean varieties suitable for planting in northern regions of China. However, much less is known about the genetic basis of plant height essential for soybean adaptation to high latitudes. Plant height in soybean is determined by the number of nodes and the length of the internodes, and is highly sensitive to the variation in the light conditions [18] . For instance, long-day photoperiods at high latitude and low blue light (LBL) under high-density planting and intercropping conditions can induce exaggerated stem elongation (ESE) syndrome, decrease the mechanical strength of the stem, result in lodging and increase susceptibility to insects and pathogens [6] , [19] , [20] . The above situations seriously constrain the improvement of soybean yield by high-density planting in high-latitude regions. It has been revealed that the blue light receptor GmCRY1s repress the LBL-induced ESE syndrome by stabilizing the bZIP transcription factors STF1 and STF2 [21] , and modulating the components of the GmCRY1-mediated signaling pathway can improve shade-tolerant traits and improve yield in soybean [22] , [23] . In this study, we identify a plant height determining gene PH13 , which has been selected in breeding soybean cultivars suitable for high latitudes. We show that a Ty1/Copia -like retrotransposon causes a truncation in PH13 H3 protein, resulting in a weaker interaction with GmCOP1a and GmCOP1b, which consequently leads to accumulation of bZIP transcription factors STF1/2 and a short plant stature. We knock out both PH13 and its paralogous gene PHP to generate a ph13php double ( phd ) mutant that displays an ideal type of shade-resistance. Our findings provide insights into the genetic basis for the breeding of modern soybeans suitable for high latitudes and offer alleles to improve soybean yield through high-density planting. Identification of plant height loci in soybean To identify genetic loci that can attenuate the extent of ESE, we phenotyped a collection of 2214 previously genotyped soybean accessions [24] for the plant height trait in a normal cultivating system in ten locations over two or three years. The best linear unbiased prediction (BLUP) for each accession was estimated to support association studies (Supplementary Data 1 ). We conducted a Genome-wide Association Study (GWAS) using 540 spring-sown improved cultivars with 3.47 million SNPs (minor allele frequency >5%) and a Transcriptome-wide Association Study (TWAS) for 488 soybean accessions (Supplementary Fig. 1a ) to identify SNPs using FarmCPU [25] and genes associated with plant height. The GWAS identified eleven plant height loci, while the TWAS identified seven genes (Supplementary Data 2 , 3 ). Of these, fourteen have not been reported previously as soybean height loci and three were refined loci associated with known candidate genes ( E2 , Dt1 and Dt2 ) [11] , [26] , [27] , validating the effectiveness of our strategy to find targeting genes (Fig. 1a, b ). Only one gene ( Glyma.13G276700 ) located on chromosome 13 was identified by both GWAS and TWAS. Hence, we named this candidate gene as Plant Height 13 ( PH13 ) for further analysis. The surrounding genetic region of PH13 has repeatedly been identified as a plant height-associated QTL in previous studies [28] , [29] , [30] , [31] , [32] , supporting a role of PH13 in regulating plant height. Fig. 1: Identification of PH13 as a major QTL for plant height in soybean. a , b Manhattan plots for GWAS (540 accessions) and TWAS (488 accessions) of soybean plant height (Supplementary Data 1 ). Each dot represents one SNP in GWAS ( a ) or gene/exon in TWAS ( b ). The p values derived from association analyses conducted using FarmCPU were log-transformed, with the gray dashed line representing the Bonferroni correction threshold for multiple test adjustments. Previously identified genes are labeled in black, and PH13 is labeled in red. The green and orange dots are arranged in alternation to distinguish them from different chromosomes. c Two types of transcripts associated with plant height variation were shown. The transcripts with normal expression levels are displayed at the top, while those with truncated expression due to the insertion of a Ty1/Copia -like retrotransposon are shown below. Five samples from each category were randomly selected and pooled for alignment visualization. d Schematic representation of the PH13 candidate gene and the insertion site of a Ty1/Copia -like retrotransposon. Solid and shaded boxes in the gene structure represent exons and UTRs, respectively. The retrotransposon diagram is shown at the bottom, with LTR representing long terminal repeats and ORF representing open reading frame. The red “G” (base 2444) represents the nonsynonymous mutation derived from exonic SNP. The red letters below denote flanking nucleotides and amino acids derived from the retrotransposon insertion. e Distribution of plant height BLUP (Best Linear Unbiased Prediction) for each haplotype. The BLUP values were calculated using the plant height data of natural populations in ten field environments over two or three years (Methods-GWAS and TWAS assays). The box plot shows the 25th to 75th percentile range, with a black line indicating the median. The whiskers extend to cover a range of 1.5 times the interquartile range, and black dots represent outliers. p values obtained from unpaired, two-tailed Student’s t -tests (Supplementary Data 7 ). Full size image The leading single nucleotide polymorphism (SNP), Gm13-37757704, identified by GWAS has a physical distance of 55,493 bp from PH13 and a linkage disequilibrium R 2 of 0.86 with the exonic SNP (Gm13-37816013) within PH13 (Fig. 1a and Supplementary Fig. 1b ). The TWAS identified the sixth exon of PH13 within this locus (Fig. 1b ). Since FarmCPU considers associated markers as covariants, which can lead to false negatives of neighboring coexpressed genes of PH13 in TWAS, we also used a mixed linear model to perform TWAS, which confirmed that PH13 is the only gene within this locus that displayed an association signal (Supplementary Fig. 1c ). A homologue of SUPPRESSOR OF PHYA is the candidate of PH13 gene The PH13 gene encoding a WD40 protein which is likely homologous to the suppressor of the phyA-105 (SPA) family protein in Arabidopsis [33] . Phylogenetic analysis indicated that PH13 is grouped closely with SPA3/4 protein (Supplementary Fig. 2a and Supplementary Data 4 ). We then transformed the 35S::PH13-3×Flag construct into the spa134 mutant [34] . The phenotypic results indicated that ectopic expression of PH13 can at least partially rescued the dwarf phenotype of the spa134 mutant at both seedling and adult vegetative stage, supporting that PH13 is homologous to the SPA family proteins (Supplementary Fig. 2b–e ). The TWAS analysis of 488 accessions revealed two forms of PH13 transcripts (Supplementary Fig. 3 ), one of which had no detectable expression from shortly after the beginning of the fifth exon to the 3’ end (Fig. 1c ). To understand the cause of this difference, we examined the coding DNA sequence (CDS) of PH13 in 1254 accessions by re-sequencing and PCR assay (Supplementary Fig. 4a, b ). Besides the exonic SNP (Gm13-37816013), a 5404 bp fragment containing two 431 bp long terminal repeats (LTRs) and a 3984 bp open reading frame (ORF) encoding Gag-protease-integrase-RT-RNaseH domains was found at the start of the fifth exon. This fragment belongs to the Ty1/Copia -like retrotransposon (Fig. 1d , Supplementary Fig. 5 and Supplementary Data 5 , 6 ). 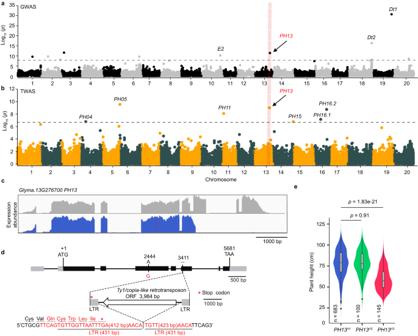Fig. 1: Identification ofPH13as a major QTL for plant height in soybean. a,bManhattan plots for GWAS (540 accessions) and TWAS (488 accessions) of soybean plant height (Supplementary Data1). Each dot represents one SNP in GWAS (a) or gene/exon in TWAS (b). Thepvalues derived from association analyses conducted using FarmCPU were log-transformed, with the gray dashed line representing the Bonferroni correction threshold for multiple test adjustments. Previously identified genes are labeled in black, andPH13is labeled in red. The green and orange dots are arranged in alternation to distinguish them from different chromosomes.cTwo types of transcripts associated with plant height variation were shown. The transcripts with normal expression levels are displayed at the top, while those with truncated expression due to the insertion of aTy1/Copia-like retrotransposon are shown below. Five samples from each category were randomly selected and pooled for alignment visualization.dSchematic representation of thePH13candidate gene and the insertion site of aTy1/Copia-like retrotransposon. Solid and shaded boxes in the gene structure represent exons and UTRs, respectively. The retrotransposon diagram is shown at the bottom, with LTR representing long terminal repeats and ORF representing open reading frame. The red “G” (base 2444) represents the nonsynonymous mutation derived from exonic SNP. The red letters below denote flanking nucleotides and amino acids derived from the retrotransposon insertion.eDistribution of plant height BLUP (Best Linear Unbiased Prediction) for each haplotype. The BLUP values were calculated using the plant height data of natural populations in ten field environments over two or three years (Methods-GWAS and TWAS assays). The box plot shows the 25th to 75th percentile range, with a black line indicating the median. The whiskers extend to cover a range of 1.5 times the interquartile range, and black dots represent outliers.pvalues obtained from unpaired, two-tailed Student’st-tests (Supplementary Data7). Three main haplotypes ( PH13 H1 -PH13 H3 ) were detected in the PH13 CDS of the 1254 accessions based on the SNPs and insertion fragment variation (Table 1 ). The haplotype 3 ( PH13 H3 ) harbors the Ty1/Copia -like retrotransposon insertion, which was predicted to produce a truncated PH13 protein (742 amino acids) lacking the 3’ part of the WD40 domain (Supplementary Fig. 6 ). This hypothesis was confirmed by immunoblot results showing that the molecular weight of PH13 H3 −3×Flag was about 10 kDa lower than that of PH13 H1 −3×Flag or PH13 H2 −3×Flag when ectopically expressed in tobacco leaves (Supplementary Fig. 7 ). Moreover, PH13 H3 accessions were found to have significantly reduced plant height compared to accessions carrying PH13 H1 and PH13 H2 under field conditions in ten field locations over two or three years (Fig. 1e and Supplementary Data 7 ), suggesting that the retrotransposon insertion in PH13 H3 is responsible for the reduction in plant height. Table 1 Three major haplotypes of PH13 identified in 1254 soybean accessions Full size table Genetic validation of PH13 function in regulating plant height Tissue-specific expression analysis showed that PH13 was expressed at a higher level in the shoots and stems compared to other tested tissues, including roots, cotyledons, unifoliate and trifoliate leaves, and flowers, supporting PH13 is involved in regulation of plant height (Supplementary Fig. 8 ). To investigate its biological role in soybean, two independent gRNAs targeting the first exon were used to generate loss-of-function mutants in the Williams 82 background (W82 H1 , harboring PH13 H1 ) using CRISPR/Cas9 technology. Three independent mutants, ph13-1 , ph13-2 , and ph13-3 , were identified with base deletion or/and insertion (Supplementary Fig. 9 ). The phenotypic results demonstrated that the loss-of-function of PH13 caused a significant dwarf phenotype with a more than 30% reduction in plant height compared to the wild type (WT) W82 H1 (Fig. 2a, b and Supplementary Fig. 10a, b ). Additionally, we generated three independent PH13 H1 −3×Flag overexpression lines ( H1-OE1/ TL1 H3 , H1-OE2/ TL1 H3 and H1-OE3/ TL1 H3 ) in the TL1 H3 background, which exhibited a significant increase in plant height (Fig. 2a and Supplementary Fig. 10d–f ). The reduction in plant height of the ph13 mutants was mainly due to a decrease in internode length (Fig. 2b and Supplementary Fig. 11 ) which was correlated with the reduced cell length (Supplementary Fig. 12 ). Moreover, the ph13 mutants showed 5 days earlier flowering time and 2 fewer nodes than W82 H1 , which also contributed to the reduction in plant height (Supplementary Figs. 10c and 11b ). Fig. 2: Genetic confirmation of PH13 as a plant height regulator. a Gross photos of the indicated lines grown under natural field conditions in the summer of Beijing. The CRISPR/Cas9-engineered mutants ph13-1 and ph13-2 are in the W82 H1 (carrying PH13 H1 ) background, and ph13-4 and ph13-6 are in the TL1 H3 (carrying PH13 H3 ) background. The PH13 H1 overexpression lines ( H1-OE1/ TL1 H3 and H1-OE2/ TL1 H3 ) are in the TL1 H3 background. Scale bar, 20 cm. b Plant height of the indicated lines as shown in a . Data are mean ± SD ( n = 10 biologically independent plants). c Plant height of the near-isogenic lines (NILs) carrying homozygous H1 (NIL H1 ) and homozygous H3 (NIL H3 ) under natural field conditions in Beijing. The NILs were derived from the hybrid combination between W82 H1 and TL1 H3 (Supplementary Fig. 13 ). The two ends of the box plot and the upper, middle, and lower box lines represent the upper edge, lower edge, median, and two quartiles of values. Data are mean ± SD ( n = 45 and 41 biologically independent plants for NIL H1 and NIL H3 , respectively). Above p values were calculated by unpaired, two-tailed Student’s t -tests. Source data are provided as a Source Data file. Full size image To assess the functionality of PH13 H3 , three independent mutants were generated using CRISPR-Cas9 technology in a Tianlong 1 backgrounds (TL1 H3 , harboring PH13 H3 with the retrotransposon insertion). Phenotypic analysis revealed that the mutants had a slightly reduced plant height of around 10% compared to the WT TL1 H3 (Fig. 2a, b ), indicating that the PH13 H3 retained some of its ability to promote plant height. In addition, near-isogenic lines (NILs) were created by crossing the W82 H1 cultivar (with an average plant height of 110 cm) with the TL1 H3 cultivar (with an average plant height of 80 cm) (Supplementary Fig. 13 ). The resulting NIL H3 plants had a significantly lower plant height than that of NIL H1 (Fig. 2c ). Collectively, these results demonstrate that PH13 functions as a plant height enhancer by promoting stem elongation and increasing node number, and the Ty1/Copia -like retrotransposon insertion had partially comprised the function of PH13 H3 in regulating plant height. PH13 H3 was artificially selected for the improvement of soybean at high latitude Given that plant height is one of the essential agronomic traits determining yield [35] , [36] , [37] , we investigated whether PH13 alleles have been utilized during soybean domestication and improvement. We analyzed the frequency and geographic distribution of the three main haplotypes among 121 accessions of G. soja , 715 landraces, and 418 improved cultivars, all with known genotypes and origin sites around the world (Supplementary Data 7 ). We found that G. soja predominantly contain PH13 H1 (99.2%) with a small amount of PH13 H2 (Fig. 3a ). Meanwhile, PH13 H3 was absent in G. soja but occurred at a low frequency of 1.4% in landraces (Fig. 3a ). Interestingly, the proportion of PH13 H3 accessions among all improved cultivars increased to 32.7%, suggesting that the PH13 H3 allele was subject to intensive artificial selection during genetic improvement. Fig. 3: The evolution and geographical distribution of PH13 different haplotypes. a The pie charts represent the percentage of accessions with different haplotypes in wild soybean, landrace, and improved cultivars. b The global geographical distribution of 1133 soybean accessions (including landrace and improved cultivars) carrying PH13 H1 , PH13 H2 , and PH13 H3 (Supplementary Data 7 ) is shown using circle. The color of the circle represents the type of germplasm, and the size of the circle represents the percentage of germplasm in respective location. Full size image The increase in the proportion of PH13 H3 in improved cultivars compared to landraces prompted us to investigate its geographical distribution in the world. We found that a large proportion of the PH13 H3 accessions were concentrated in high-latitude regions, while the other two haplotypes were dispersed more evenly (Fig. 3b ). This geographical bias was further analyzed in China where the proportion of PH13 H3 among all cultivars increased from near zero in the lower latitude regions (below 40°N) to 48.7% in the higher latitude regions (above 40°N) (Supplementary Fig. 14a–d ). Out of 78 cultivars carrying PH13 H3 , 76 were located in higher latitude regions (Supplementary Fig. 14e ), demonstrating that the PH13 H3 allele has been used successfully in breeding programs to improve soybean adaptation in high latitudes. The protein products of PH13 H3 have reduced binding affinity with two GmCOP1 E3 ubiquitin ligases PH13, being a SPA homologous protein in soybean, possesses a conserved kinase domain, coiled-coil domain, and WD40 domain, while the protein products of PH13 H3 lacks the intact WD40 domain (Supplementary Figs. 6 and 7 ). In order to assess the impact of the retrotransposon insertion on PH13’s function, we conduced RT-qPCR analysis on W82 H1 and TL1 H3 cultivars. The results revealed that the insertion did not affect the transcription of the sequence before the insertion site, but abolished the transcription of the carboxyl terminus (Fig. 4a, b ), which is consistent with the expression patterns observed in natural population (Fig. 1c ). Further analysis of the subcellular location of different PH13 haplotypes showed that the retrotransposon did not alter the location of the truncated PH13 H3 protein in both nucleus and cytoplasm (Supplementary Fig. 15 ). Fig. 4: Comparison of transcripts and protein activities of different haplotype of PH13 . Transcript levels of PH13 H1 in W82 and PH13 H3 in TL1 respectively, were measured using primers detecting the expression of exon 3 ( a ) and 3’UTR ( b ). c Transcript levels of PH13 H1 , GmCOP1a , and GmCOP1b in W82. The second trifoliate leaves of 20-day-old seedlings grown under long-day conditions were collected at 4-hour intervals for RT-qPCR analysis. Data are mean ± SD ( n = 3 biologically independent replicates) calculated relative to GmActin . d Protein structure of each haplotype. aa, amino acids. e Auxotrophic assays showing the interactions between different PH13 haplotypes with GmCOP1s. Yeast cells transformed with indicated constructs were selected on -LW (lacking Leu and Trp) or -LWHA (lacking Leu, Trp, His and Ade) medium. AD, GAL4 activation domain; BD, GAL4 DNA-binding domain. f Co-Immunoprecipitation (Co-IP) assay showing the interaction between each PH13 haplotype with GmCOP1b in tobacco leaves. The indicated constructs were co-transformed into tobacco which were then incubated at 25 °C in dark for 12 h and grown under white light (WL, 80 μmol m −2 s −1 ) for 36 h. The immunoprecipitates were detected using anti-GFP (at a 1:2500 dilution) and anti-Flag (at a 1:2500 dilution) antibodies, respectively. Empty vector ( 35 S::YFP ) was used as a negative control. Numbers at bottom represent the relative IP efficiency, calculated as (IP-PH13/Input-PH13)/(IP-GmCOP1b/Input-GmCOP1). A representative result of three independent replicates is shown. g Immunoblots showing STF1/2 protein levels in the NIL H1 and NIL H3 lines under diurnal conditions. The first trifoliate leaves of 15-day-old seedlings grown under long-day condition were collected at 4-hour intervals. The membrane was probed with the anti-STF1/2 antibody (at a 1:1000 dilution), stripped, and then probed with the anti-HSP70 antibody (at a 1:10,000 dilution). The asterisk indicates a non-specific band. h The relative expression level of STF1/2 proteins represented by REU (Relative Expression Unit) was calculated by the formula [STF1/2] / [HSP70], in which ‘STF1/2’ and ‘HSP70’ indicate the digitized band intensity of STF1/2 or HSP70 in each sample collected at respective time point. The REU of STF1/2 in NIL H1 at ZT0 was arbitrarily set to 1. Data are shown as means ± SD of three biological replicates (Supplementary Fig. 18 ). Source data are provided as a Source Data file. Full size image The SPA family is known to suppress photomorphogenesis, as part of a complex with COP1, serving as E3 ubiquitin ligases to target multiple transcription factors for degradation in Arabidopsis [38] , [39] , [40] . A previous study showed that two soybean COP1 orthologs, GmCOP1a and GmCOP1b, play a pivotal role in controlling plant height in soybean [22] . Here we found that the diurnal transcription pattern of PH13 is in line with that of GmCOP1a and GmCOP1b in soybean, peaking at dawn and declining at dusk (Fig. 4c ), suggesting that PH13 may act as an evolutionarily conserved factor to form a complex with these GmCOP1s to degrade target proteins in soybean. This prompted us to investigate whether the retrotransposon affects the interaction of PH13 with GmCOP1s. Yeast-two hybrid (Y2H) and Co-Immunoprecipitation (Co-IP) experiments revealed that these GmCOP1s strongly interact with PH13 H1 and with PH13 H2 but weakly with PH13 H3 (Fig. 4d–f and Supplementary Fig. 16 ). Domain-specific Y2H assays indicated that PH13 interacts with GmCOP1b via their coil-coil domains, but the WD40 domain of PH13 can significantly enhance their interaction strength (Supplementary Fig. 17a–c ). These results together demonstrate that the absence of the WD40 domain in PH13 H3 reduces the interaction strength between PH13 and GmCOP1s in soybean. PH13 and its paralogue PHP function together to decrease STF1/2 abundance Given previous evidence that GmCOP1s mediate the degradation of STF1/2 transcription factors which are homologous to Arabidopsis HY5 and responsible for inhibiting stem elongation in legume [21] , [22] , [41] , [42] , we sought to determine whether the altered interaction of the truncated PH13 with GmCOP1s affects the accumulation of STF1/2 proteins. Our results showed that the overall protein levels of STF1/2 increased by 39–144% during a diurnal cycle in the NIL H3 line compared to NIL H1 line grown under long day condition in growth chamber (Fig. 4g, h and Supplementary Fig. 18 ). This indicates that the insertion retrotransposon in NIL H3 enhances the accumulation of STF1/2. Additionally, the pattern of STF1/2 protein accumulation, which peaked in the middle of the day (Fig. 4h ), was opposite to that of the GmCOP1s and PH13 transcripts peaking at night (Fig. 4c ). This suggests that the GmCOP1s-PH13 E3 ligases play a role in modulating the abundance of the STF1/2 protein in response to photoperiod. While the abundance of the STF1/2 protein increased in the NIL H3 line, its expression pattern remained unchanged and its level still decreased during the night period (Fig. 4h and Supplementary Fig. 18 ), suggesting a possibility that some homologous genes may act redundantly or additively with PH13 to regulate the degradation of STF1/2. Indeed, the soybean genome contains a PH13 paralogue Glyma.12G224600 , which we hereafter name PHP , encoding a protein with 96.6% amino acid similarity to PH13 (Supplementary Figs. 2a and 19 ). We then generated multiple php and ph13/php double ( phd ) mutant lines using CRISPR/Cas9 technology in the TL1 H3 background (Supplementary Fig. 20 ). Phenotypic analysis revealed a progressive reduction in plant height in the order of TL1 H3 , ph13 , php , and phd (Supplementary Fig. 21 ), indicating that the PH13 and PHP genes act cooperatively in regulating plant height. We observed at least 3-fold increase in STF1/2 protein abundance in the phd-1 mutant compared to the WT TL1 H3 (Supplementary Fig. 22 ) especially at night. To verify whether PH13 and PHP act as upstream regulators of STF1/2 , we crossed the phd-1 mutant with the stf1/2 mutant [43] (Supplementary Fig. 23a ). Phenotypic assessment showed partial rescue of the dwarf phenotype of the phd-1 mutant by the stf1/2 mutant (Supplementary Fig. 23b, c ), suggesting that STF1/2 act as downstream targets of PH13 and PHP to influence plant height. PH13 and PHP redundantly regulate LBL-induced exaggerated stem elongation Considering that low blue light (LBL) triggers degradation of STF1/2 and leads to ESE syndrome in soybean [21] , we hypothesize that the increased abundances of STF1/2 in the ph13 , php and phd mutants might result in an appropriate extent of stem elongation for high yield under shade conditions. To test this, we compared the performance of each mutant line with the WT TL1 H3 in response to simulated shade regimes (Fig. 5a and Supplementary Fig. 24 ). Our results showed that LBL efficiently induced ESE syndrome in the ph13 and php mutants as well as in TL1 H3 , but not in the phd mutant (Fig. 5b ). Fig. 5: CRISPR/Cas9 targeting of the PH13 gene and its paralog ( PHP ) abolished the LBL induced ESE and enhanced yield under different planting densities. a Representative images of the php-1 , ph13-4 , and phd-1 mutants and WT TL1 under different light regimes. Seedlings were grown under white light (WL), LBL, and WL plus far-red (L R:FR) for 15 days after de-etiolation with white light under long-day conditions. The intensity of photosynthetically active radiation (PAR) was maintained at approximately 500 μmol m −2 s −1 (Supplementary Fig. 24 ). Scale bar corresponds to 20 cm. b Plant height and internode length of the indicated lines shown in a . Data are means ± SD ( n = 6 biologically independent plants for b ). 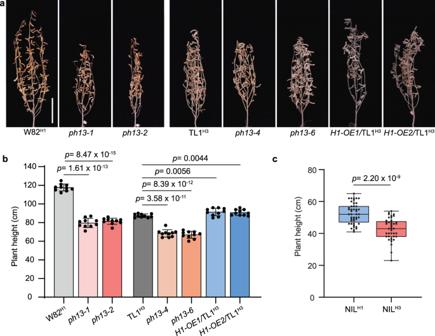Fig. 2: Genetic confirmation ofPH13as a plant height regulator. aGross photos of the indicated lines grown under natural field conditions in the summer of Beijing. The CRISPR/Cas9-engineered mutantsph13-1andph13-2are in the W82H1(carryingPH13H1) background, andph13-4andph13-6are in the TL1H3(carryingPH13H3) background. ThePH13H1overexpression lines (H1-OE1/TL1H3andH1-OE2/TL1H3) are in the TL1H3background. Scale bar, 20 cm.bPlant height of the indicated lines as shown ina. Data are mean ± SD (n= 10 biologically independent plants).cPlant height of the near-isogenic lines (NILs) carrying homozygous H1 (NILH1) and homozygous H3 (NILH3) under natural field conditions in Beijing. The NILs were derived from the hybrid combination between W82H1and TL1H3(Supplementary Fig.13). The two ends of the box plot and the upper, middle, and lower box lines represent the upper edge, lower edge, median, and two quartiles of values. Data are mean ± SD (n= 45 and 41 biologically independent plants for NILH1and NILH3, respectively). Abovepvalues were calculated by unpaired, two-tailed Student’st-tests. Source data are provided as a Source Data file. Different letters indicate statistically significant differences as determined by two-way ANOVA with two-sided Tukey test at the 0.05 level. c Gross photos of the WT TL1 and phd-1 mutant plants (upper panel, Scale bar, 20 cm) and the whole seeds (bottom panel, Scale bar, 2 cm) produced by respective plant grown with 30 cm, 20 cm, 10 cm, or 5 cm plant space, respectively. Statistical analysis of the plant height ( d ), grain yield per plant ( e ), and grain yield per plot ( f ) of each indicated line. Data are means ± SD ( n = 20 biologically independent plants for d and e ; n = 3 biologically independent field plots for f ). p values are from unpaired, two-tailed Student’s t -tests. Source data are provided as a Source Data file. Full size image The blue light receptor, GmCRY1s, was observed to mainly mediated LBL-induced shade avoidance syndrome (SAS) in soybean [21] . Next, we crossed the CRISPR-Cas9-engineered Gmcry1s quadruple ( Gmcry1s-qm ) mutant [21] displaying constitutive ESE syndrome, with the phd-1 mutant carrying stocky phenotype, to obtain the phd-1/Gmcry1s-qm sextuple mutant (Supplementary Fig. 25a ). We found that the phd mutations partially rescued the ESE syndrome of the Gmcry1-qm mutant in field conditions (Supplementary Fig. 25b–d ), suggesting that PH13 and PHP may be genetically downstream of GmCRY1s in regulating of LBL-induced stem elongation. Furthermore, the phd mutant was found to display a semi-dwarf phenotype due to decreased internode length, rather than reduced node number in comparison with TL1 H3 , under LBL conditions (Fig. 5b ). Moreover, the phd mutant was distinguished by its thicker stem compared to other lines under all light conditions (Fig. 5a and Supplementary Fig. 26 ). Collectively, these results demonstrate that the phd mutant is characterized by ideal shade-resistant traits, which may be advantageous for high-density planting or intercropping at high latitudes. Knockout of PH13 and PHP enable TL1 H3 to adapt to high latitudes Generally, the allopatric planting of lower-latitude soybean cultivars in higher-latitude region can induce excessive stem growth and lead to severe lodging due to the extended vegetative phase (Supplementary Fig. 27 ). To verify if the phd mutants could be utilized to enhance the adaptability of cultivars to higher latitudes, we conducted field trails in Changchun (125°19′E, 43°53′N) and Xuchang (104°31′E, 34°10′N) and compared the extent of stem elongation between the phd mutants and TL1 H3 (Supplementary Fig. 28a, b ). The results showed that the phd mutant had a lower fold change in stem elongation between the two latitudes than TL1 H3 (Supplementary Fig. 28c ). Moreover, the phd mutants had a lower lodging rate, earlier maturity time, more branches, and a higher pod number per plant than the ph13 , php mutants, and WT TL1 H3 (Supplementary Fig. 29 ). In addition, we observed that the phd mutants exhibit a larger root system at seedling stage in growth chamber and at maturity stage in Beijing field conditions (Supplementary Fig. 30 ). Above results further suggesting the potential of using the phd mutant to improve the adaptability of soybean to high-latitude regions. The phd mutants is suitable for high-density planting or intercropping We evaluated the yield performance of the phd mutants at different planting densities (30 cm, 20 cm, 10 cm, and 5 cm plant space, equivalent to approximately 67,000, 100,000, 200,000, and 400,000 plants per hectare) in Changchun (Supplementary Fig. 31 ). The results showed that the main stem length of TL1 H3 increased with the increase of planting density (IPD), resulting in severe lodging at all planting densities, whereas the phd mutants were insensitive to IPD and no lodging occurred (Fig. 5c, d and Supplementary Figs. 31c , 32c ). While the yield per plant decreased with the IPD for TL1 H3 , the phd mutants consistently outperformed it (Fig. 5e and Supplementary Fig. 32 ). The plot yields of the phd mutants increased significantly in response to the IPD, while remaining unchanged or even decreased for TL1 H3 (Fig. 5f ). Moreover, the phd mutant lines showed better performance than a local elite cultivar Jiyu202 (JY202) at high planting density (400,000 plants per hectare) (Supplementary Fig. 33a ). Despite being shorter than JY202, the phd mutants did not display any difference in node number (Supplementary Fig. 33d ). 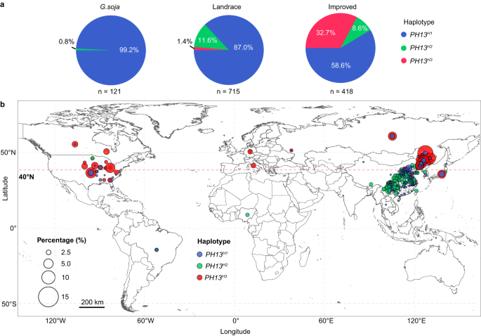Fig. 3: The evolution and geographical distribution ofPH13different haplotypes. aThe pie charts represent the percentage of accessions with different haplotypes in wild soybean, landrace, and improved cultivars.bThe global geographical distribution of 1133 soybean accessions (including landrace and improved cultivars) carryingPH13H1,PH13H2, andPH13H3(Supplementary Data7) is shown using circle. The color of the circle represents the type of germplasm, and the size of the circle represents the percentage of germplasm in respective location. Additionally, the phd mutants had a thicker stem, lower lodging rate, more branches, more pods per plant, as well as a 15.8% increase in grain yield per plant compared to JY202 (Supplementary Fig. 33b–h ). Furthermore, we evaluated the shade-tolerant ability of the phd mutants under a maize-soybean relay intercropping system at even higher latitudes in Harbin (127°50’E, 45°70’N). The results showed that the phd mutants were significantly shorter than TL1 H3 as well as LK317 and LK18-842 (Supplementary Fig. 34a–c ), two elite cultivars used for maize-soybean intercropping in Harbin. Moreover, lodging did not occur in the phd mutants, while nearly 100%, 40% and 80% lodging rates were observed in TL1, LK317 and LK18-842, respectively (Supplementary Fig. 34d ). The plot yield of the phd mutants was at par with that of LK317 and LK18-842 (Supplementary Fig. 34e ). These results together demonstrate that knockout of PH13 and PHP can improve the adaptability of TL1 H3 , a cultivar of mid latitude, to higher latitude for high density planting or intercropping. The global demand for soybeans is expected to continue rise in the future due to several factors such as the rising consumption of meat and soy-based health products, growing populations, and a more favorable policy of biofuels. Currently, the majority of soybean cultivation is located in mid to low latitude countries, including the United States, Brazil, and Argentina, which together contribute 80% of the total global yield [44] . Thus, there present a great opportunity for soybean production in high-latitude regions, such as Canada, northern US, northern China, and Russia, which could potentially serve as the primary source of increased soybean production in the future. However, high-latitude regions have short frost-free periods and a long-day photoperiod, which can lead to excessive stem elongation and lodging. Those require the development of soybean varieties with a shorter growth period and reduced plant height. In this study, a natural variant of the PH13 gene ( PH13 H3 ) was identified that has been unintentionally utilized in the breeding of modern soybean varieties in northern latitude regions. The underlying mechanism of the reduced plant height was determined to be the insertion of the Ty1/Copia -like retrotransposon in the PH13 gene, causing a partial loss of the WD40 domain in the PH13 protein (Fig. 4d ) and weakening its interaction with GmCOP1s and allowing the accumulation of downstream transcription factors STF1/2 (Fig. 4g, h ), which subsequently inhibit internode elongation. The interaction between PH13 and GmCOP1b is mediated by their coil-coil domains, and enhanced by the WD40 domain of PH13. This is likely different from Arabidopsis , where the interaction between SPA1 (a homologous protein of SPA3/4 and PH13) and COP1 is also mediated by their coil-coil domains, and the absence of the WD40 domain of SPA1 does not impair the interaction with COP1 [45] . Furthermore, COP1 and SPAs have been reported to co-localize and function together within the nucleus in Arabidopsis [46] , [47] , whereas PH13 lacks an NLS (Nuclear Localization Signal) and is uniformly distributed in both the nucleus and cytoplasm (Supplementary Figs. 15 and 19 ). This suggests that PH13 may be involved in a distinct mechanism for regulating soybean growth and development. Although the PH13 H3 allele has been strongly selected in northern latitudes, its ability to reduce plant height may be insufficient and needs to be combined with early flowering loci to suit the environmental requirements of higher latitude regions [14] , [48] , [49] . This is evidenced by the TL1 H3 cultivar, which harbors the PH13 H3 haplotype but exhibits severe ESE and lodging in the northern regions (Fig. 5c and Supplementary Fig. 27 ). To address this problem, the PH13 gene and its paralog gene PHP were simultaneously eliminated to produce the phd mutants in TL1 H3 background, which exhibit both reduced plant height and early maturity suitable for planting at high latitudes (Fig. 5d and Supplementary Fig. 29f ). Additionally, many current soybean variates in the north latitudes are not suitable for high-density planting and soybean-maize intercropping which can exacerbate the problem of lodging caused by long-day photoperiods [20] , [50] . Low blue light (LBL) is the main shade avoidance signal that induces the ESE syndrome in soybean [21] . The phd mutant is insensitive to LBL and lodging resistant (Fig. 5a, b ), thus significantly increasing yield under high-density planting conditions at high latitudes (Fig. 5e, f ). Moreover, the phd mutations can also benefit intercropping by reducing the lodging-induced yield reduction (Supplementary Fig. 34d, e ). Although the phd mutant in the TL1 background exhibited lower yield potential compared to the elite cultivars LK317 and LK18-842 in Northern China under norm planting conditions, it displayed a lower lodging rate and a similar grain yield potential relative to the elite cultivars LK317 and LK18-842 under maize-soybean relay intercropping conditions. In conclusion, this study identified a pair of plant height regulatory genes that can improve soybean adaptation to high latitude and provided a strategy for breeding high-yield varieties suitable for dense planting and intercropping at high latitudes (Fig. 6 ). Fig. 6: A proposed working model of PH13 and PHP for breeding of elite cultivar suitable for high density planting in high latitudes. The insertion of the Ty1/Copia -like retrotransposon in the PH13 H3 gene attenuates the interaction between PH13 and GmCOP1s and increases the abundance of STFs protein, resulting in a stocky architecture in the natural population. The soybean accessions harboring PH13 H3 were selected during improvement and utilized by modern breeders at high latitude. The phd double mutants (harbors mutation in both PH13 and PHP ) display excellent shade traits under high-density planting conditions, which can be further utilized to improve the yield at high latitudes. Full size image Plant materials and growth conditions The high-quality genome sequences of 2214 accessions have been published before [24] . Among these materials, 540 improved cultivars with phenotype data were utilized for GWAS, resulting in the discovery of an association between genotype and phenotype variation. Furthermore, TWAS analysis uncovered an association between gene between gene expression and phenotype variation in 488 soybean accessions that possessed both phenotype and expression data. Detailed information of these materials is available in Supplementary Data 1 . In this study, the soybean ( Glycine max (L.) Merr.) cultivar Tianlong 1 (TL1) and Williams 82 (W82) served as control groups to generate transgenic lines. To evaluate plant height, we cultivated WT, ph13 , php , and phd mutants, as well as PH13 overexpression lines under long day conditions (16 h light/8 h dark at 26 °C) in a controlled growth chamber. For the field experiment, the aforementioned transgenic materials were grown naturally from May to October in three different locations: the Institute of Crop Science, Chinese Academy of Agricultural Science, Beijing (116°23′E, 39°54′N), Jilin Agricultural University, Changchun (125°19′E, 43°53′N), Beidahuang KenFeng Seed Co., Ltd, Harbin (127°50’E, 45°70’N). To assess the plant density effects, four treatments with three replicates each were conducted in Changchun. Seeds were sown in May with varying plant spacings (30 cm, 20 cm, 10 cm, and 5 cm, resulting in plant densities of 66,700, 100,000, 200,000, and 400,000 plants per hectare, respectively). The plots were organized in 3 m long rows with 0.5 m between each row, covering a total area of 7.5 square meters. Harvesting was performed in October 2021. For the maize-soybean relay intercropping experiments, seeds were sown in early May in Harbin, with a row-to-row distance of 40 cm between maize plants, and between soybean plants, and 60 cm between maize and soybean. The soybean was spaced 5 cm apart in rows of 5 m in length (equivalent to 400,000 plants per hectare), while the maize was spaced 10 cm apart in rows of 5 m in length. To maintain uniformity, all lines under different densities were manually planted with 3 seeds per hole. Once the seeds geminated and the unifoliate leaf fully unfolded, only one healthy seedling was retained per hole. Failed seedlings were removed and replaced with a healthy seedling of same genotype via transplanting to maintain uniformity. The plot size was 19.7 square meters, and two biological replicates were conducted for each experimental material. Harvesting was performed in October 2022. At the R8 stage (when 95% of pods had reached maturity), the following agronomic traits were measured: plant height, length of the internodes, number of branches, node number, height of the center of gravity point, pods per plant, lodging rate, grain yield per plant, and grain yield per plot were measured. Soybean lodging resistance was evaluated based on the height of the center of gravity point, a measure of the balance point at which mature plants were placed in a horizontal position. At least ten randomly selected plants within each plot were included in the phenotypic analysis for each measured trait. GWAS and TWAS assays A panel of 857 soybean accessions (Supplementary Fig. 1a ) were genotyped and phenotyped for plant height for association analysis in a previous study [24] . The plant materials were planted in ten different environments and evaluated for a minimun of two years to record plant height data. These environments included Harbin (45°45’N, 126°41’E) from 2017 to 2019, Changchun (43°88’N, 125°25’E) in 2018 and 2019, Tonghua (41°74’N, 125°94’E) from 2017 to 2019, Shijiazhuang (38°05’N, 114°52’E) in 2018 and 2019, Liaocheng (36°46’N, 115°99’E) from 2017 to 2019, Xuzhou (34°27’N, 117°19’E) in 2018 and 2019, Nanjing (31°05’N, 118°78’E) in 2018 and 2019, Hefei (31°88’N, 117°17’E) in 2018 and 2019, Wuhan (30°58’N, 114°32’E) in 2018 and 2019, and Nanchang (28°32′N, 116°1’E) from 2017 to 2019. Each cultivar was planted in a 1.8 m × 0.8 m plot with two rows and a spacing of 10 cm between seedlings in each row. The soybean lines’ plant height Best Linear Unbiased Predictions (BLUPs) were calculated using a mixed linear model ( 1 ) [51] . Here, Y represents the observed plant height, X is the fixed effects, β is the vector of fixed effect coefficients, Z is the random effects, u is the random effect coefficients, and e is the residual errors. Y=Xβ+Zu+e
 (1) In the model, the fixed effect represents the mean plant height across all lines, locations, and years. Random effects account for variations within each line, location, year, and their interactions (Line: Location and Line: Year). To address incomplete data in some lines across experimental trials, both Year and Location were treated as random effects. The re-sequencing of 2214 soybean accessions generated 8,785,134 SNPs, which were imputed by beagle [24] . After filtering the imputed SNPs for a minor allele frequency of >5% among the genotyped and phenotyped 540 soybean accessions, the remaining 3,469,934 SNPs were retained and used for plant height GWAS. The GWAS was performed using the fixed and random model Circulating Probability Unification (FarmCPU) [25] , with population structure controlled by the first three components from SNPs principal components analysis (PLINKv1.90) [52] . The resulted p -values were adjusted with Bonferroni correction at a level of α = 0.05, resulting in a cutoff of 1.44E−08. A natural panel (PRJCA014188) of previously published RNA-Seq data from tissues above cotyledonary node at the V2 stage was employed for TWAS. A total of 488 soybean accessions, possessing both expression and phenotype data, were included in the analysis and underwent TWAS using FarmCPU [25] . Genes and exons with an average Transcripts Per Million (TPM) > 0.1 were considered to be expressed as described by Li et al. [53] . Population structure was controlled by the first three components from the expression principal components analysis. The resulting p -values were adjusted using Bonferroni correction at a level of α = 0.05. 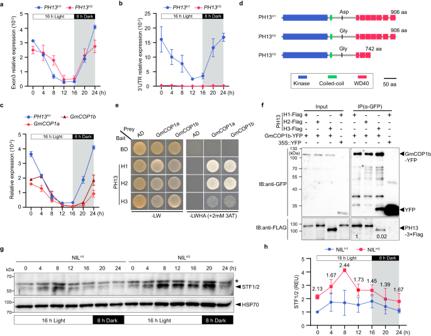Fig. 4: Comparison of transcripts and protein activities of different haplotype ofPH13. Transcript levels ofPH13H1in W82 andPH13H3in TL1 respectively, were measured using primers detecting the expression of exon 3 (a) and 3’UTR (b).cTranscript levels ofPH13H1,GmCOP1a, andGmCOP1bin W82. The second trifoliate leaves of 20-day-old seedlings grown under long-day conditions were collected at 4-hour intervals for RT-qPCR analysis. Data are mean ± SD (n= 3 biologically independent replicates) calculated relative toGmActin.dProtein structure of each haplotype. aa, amino acids.eAuxotrophic assays showing the interactions between different PH13 haplotypes with GmCOP1s. Yeast cells transformed with indicated constructs were selected on -LW (lacking Leu and Trp) or -LWHA (lacking Leu, Trp, His and Ade) medium. AD, GAL4 activation domain; BD, GAL4 DNA-binding domain.fCo-Immunoprecipitation (Co-IP) assay showing the interaction between each PH13 haplotype with GmCOP1b in tobacco leaves. The indicated constructs were co-transformed into tobacco which were then incubated at 25 °C in dark for 12 h and grown under white light (WL, 80 μmol m−2s−1) for 36 h. The immunoprecipitates were detected using anti-GFP (at a 1:2500 dilution) and anti-Flag (at a 1:2500 dilution) antibodies, respectively. Empty vector (35S::YFP) was used as a negative control. Numbers at bottom represent the relative IP efficiency, calculated as (IP-PH13/Input-PH13)/(IP-GmCOP1b/Input-GmCOP1). A representative result of three independent replicates is shown.gImmunoblots showing STF1/2 protein levels in the NILH1and NILH3lines under diurnal conditions. The first trifoliate leaves of 15-day-old seedlings grown under long-day condition were collected at 4-hour intervals. The membrane was probed with the anti-STF1/2 antibody (at a 1:1000 dilution), stripped, and then probed with the anti-HSP70 antibody (at a 1:10,000 dilution). The asterisk indicates a non-specific band.hThe relative expression level of STF1/2 proteins represented by REU (Relative Expression Unit) was calculated by the formula [STF1/2] / [HSP70], in which ‘STF1/2’ and ‘HSP70’ indicate the digitized band intensity of STF1/2 or HSP70 in each sample collected at respective time point. The REU of STF1/2 in NILH1at ZT0 was arbitrarily set to 1. Data are shown as means ± SD of three biological replicates (Supplementary Fig.18). Source data are provided as a Source Data file. However, a potential issue of the FarmCPU model is its integration of leading markers as co-variants, which can remove co-expressed and result in false-negative TWAS results. To address this issue, TWAS was also conducted using a compressed mixed linear model implemented in GAPIT [54] , [55] . DNA isolation and detection of PH13 haplotype The DNA of 1254 accessions (out of 2214 genome sequenced accessions) were extracted from leaves individually using the modified CTAB method [56] . The status of a SNP (A or G) located 2444 bp downstream of the translation start site (TSS) was determined using the resequencing data [24] . To identify the insertion of the Ty1/Copia -like retrotransposon, three primers were designed for polymerase chain reaction (PCR) detection (Supplementary Data 8 ). The presence of the fragment insertion was confirmed by agarose gel electrophoresis. Construction of near isogenic lines The creation of a pair of near-isogenic lines (NILs), consisting of NIL H1 and NIL H3 , was achieved through the crossbreeding of Williams82 carrying Hap1 (W82 H1 ) and Tianlong1 carrying Hap3 (TL1 H3 ). In the progenies of the F7 generation, a heterozygous line at the PH13 gene was selected, and the F8 generation segregating groups, carrying homozygous H1 (NIL H1 ) and homozygous H3 (NIL H3 ) were used for phenotypic analysis (Supplementary Fig. 13 ). Segregation of the PH13 haplotypes was analyzed by PCR using the three primers designed for the Ty1/Copia -like retrotransposon insertion, and confirmed through agarose gel electrophoresis. Seeds heterozygous in the targeted region from the F8 generation were grown in the phytotron or field, and the plant height phenotypes of the segregating progeny were recorded at the R8 stage. Plasmid construction and plant transformation To generate CRISPR/Cas9 engineered mutants, multiple gRNAs were designed for each gene on the basis of their specificity and off-target effects using the CRISPR direct website ( http://crispr.dbcls.jp/ ) [57] . CRISPR/Cas9 vectors were constructed using multiple target gRNA for each gene in order to improve editing efficiency and minimize off-target effects [16] . The editing efficiency of each construct was evaluated using the soybean hairy root system [58] , and at least two vectors independently with high editing efficiency for each gene were selected for soybean transformation. The selected CRISPR/Cas9 vectors were introduced into the Agrobacterium tumefaciens strain EHA105 through electroporation, and then separately transformed into W82 H1 and TL1 H3 using the cotyledon-node method [59] . To construct the overexpression vector, the coding DNA sequence (CDS) of PH13 was amplified from cDNA derived from young W82 H1 seedlings via PCR. The CDS was then cloned into the 35 S::3×Flag vector with an XhoI site, which was constructed based on the pFGC5941 plasmid containing the ( 2×35 S )-( 3×Flag )- NOS cassette inserted between EcoRI and HindIII sites [60] . The newly generated construct, 35 S::PH13 H1 −3×Flag , was then introduced into Agrobacterium strain EHA105 for the transformation of TL1 [16] . Additionally, the 35 S::PH13 H1 −3×Flag vector was introduced into the Arabidopsis spa134 mutant [34] for ectopic expression. The applied primers were listed in the Supplementary Data 8 . RNA extraction and gene expression analysis To investigate the transcriptional dynamics of PH13 in different genotypes and assess the co-expression of PH13 and GmCOP1s , we grew W82 H1 and TL1 H3 separately under long-day conditions for 20 days. The second fully expanded trifoliolate leaves were harvested every 4 hours over a day. Two pairs of primers were designed for qPCR to detect the expression levels of different PH13 alleles, one targeting exon 3, and the other targeting the 3’UTR. Total RNA was extracted using Trizol Reagent (TIANGEN), and then treated with DNase. A reverse transcription kit (TransGen Biotech) was used to synthesized cDNA from 3 μg of total RNA in a 20 μl reaction. RT-qPCR was performed on 384-well optical plate using the ABI Q7 equipment and the SYBR Green RT-PCR kit (Vazyme Biotech). All primers used for the indicated genes were listed in the Supplementary Data 8 . Three independent biological replicates were carried out for each sample. Multiple alignment and phylogenetic analysis The protein sequences of AtSPAs (AtSPA1 AT2G46340, AtSPA2 AT4G11110, AtSPA3 AT3G15354, AtSPA4 AT1G53090) were retrieved from TAIR ( https://www.arabidopsis.org/index.jsp ). Homologous SPA protein sequences were sourced from Phytozome ( https://phytozome.jgi.doe.gov/pz/portal.html ), with the list of the homologous SPA protein sequences utilized in this study outlined in Supplementary Data 4 . The amino acid sequences of the SPA proteins and their homologous proteins were aligned by ClustalW in MEGA7 with manually adjustments. The phylogenetic tree was constructed using the neighbor joining method in MEGA7 software. Subcellular location in protoplasts To investigate the subcellular location of different PH13 haplotype proteins, the CDSs of PH13 H1 , PH13 H2 , and PH13 H3 were inserted into the pA7-YFP vector at the BamHI and SmaI sites using the In-Fusion system, respectively (TransGen Biotech). The resulting PH13 Hs -YFP transient expression constructs were driven by the 35 S promoter. Control experiments were performed utilizing the empty pA7-YFP vector. Additionally the GmMYB29-RFP fusion protein was employed as a nucleus marker [61] . The plasmids were transformed into Arabidopsis mesophyll protoplasts and the resultant subcellular localization was imaged using a Zeiss LSM980 confocal laser scanning microscope. ZEN 2009 Light Edition software was used to process the images. All primers used for vector construction were listed in the Supplementary Data 8 . Yeast two-hybrid assays The yeast two-hybrid assays were conducted following the manufacturer’s instructions (Yeast Handbook Clontech). The CDSs of PH13 H1 , PH13 H2 , PH13 H3 , PH13N , PH13CT , PH13cc , and PH13WD40 were individually cloned in frame with the GAL4 DNA binding domain in the bait vector pGBKT7 (Clontech, catalog no. 631604). While the CDSs of GmCOP1a and GmCOP1b were similarly fused with the GAL4 transcription activation domain in the prey vector pGADT7 (Clontech, catalog no. K1612-1). The bait and prey plasmids were then co-transformed into the yeast strain Saccharomyces cerevisiae AH109 (Clontech). The transformed yeast cells were grown on SD/-Leu-Trp (-LW) minimal medium. Positive clones were selected and grown on SD/-His-Leu-Trp-Ade (-LWHA) selection medium at 30 °C for 3–5 days to evaluate protein interactions. The β-galactosidase activity assay was performed as previously reported [62] . Briefly, yeast colonies were selected and cultured at 180 rpm and 28 °C in an incubator until the optical density (OD600) of the culture reached 0.1 in a 10 mL flask containing 4 ml of SD medium (-Leu/-Trp). 2 mL of yeast culture was then transferred into 8 mL YPDA culture solution and cultured at 180 rpm at 28 °C until the OD600 reached 0.5-0.8 prior to the β-galactosidase assay. The relative bait-prey interaction was presented as β-gal units (2), where T is the response time (min) and V represents 0.1 × concentration factor. β-gal  units=1000×OD578/(T×V×OD600)
 (2) Co-immunoprecipitation assays To evaluate the strength of interactions between different haplotypes of PH13 and GmCOP1b, a co-immunoprecipitation (Co-IP) assay was conducted in N. benthamiana . The PH13 H1 -Flag , PH13 H2 -Flag or PH13 H3 -Flag constructs were co-transformed with the GmCOP1b-YFP construct as indicated into N. benthamiana leaves. 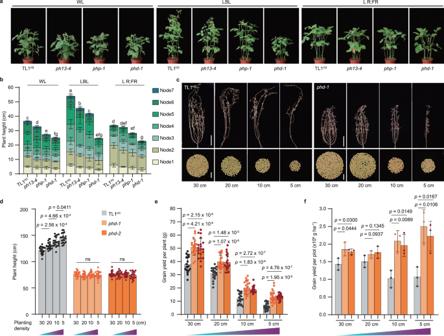Fig. 5: CRISPR/Cas9 targeting of thePH13gene and its paralog (PHP) abolished the LBL induced ESE and enhanced yield under different planting densities. aRepresentative images of thephp-1,ph13-4, andphd-1mutants and WT TL1 under different light regimes. Seedlings were grown under white light (WL), LBL, and WL plus far-red (L R:FR) for 15 days after de-etiolation with white light under long-day conditions. The intensity of photosynthetically active radiation (PAR) was maintained at approximately 500 μmol m−2s−1(Supplementary Fig.24). Scale bar corresponds to 20 cm.bPlant height and internode length of the indicated lines shown ina. Data are means ± SD (n= 6 biologically independent plants forb). Different letters indicate statistically significant differences as determined by two-way ANOVA with two-sided Tukey test at the 0.05 level.cGross photos of the WT TL1 andphd-1mutant plants (upper panel, Scale bar, 20 cm) and the whole seeds (bottom panel, Scale bar, 2 cm) produced by respective plant grown with 30 cm, 20 cm, 10 cm, or 5 cm plant space, respectively. Statistical analysis of the plant height (d), grain yield per plant (e), and grain yield per plot (f) of each indicated line. Data are means ± SD (n= 20 biologically independent plants fordande;n= 3 biologically independent field plots forf).pvalues are from unpaired, two-tailed Student’st-tests. Source data are provided as a Source Data file. 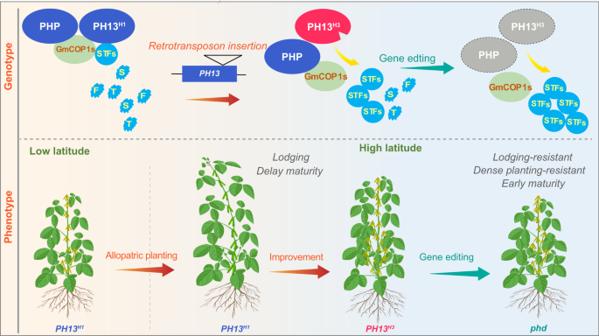Fig. 6: A proposed working model ofPH13andPHPfor breeding of elite cultivar suitable for high density planting in high latitudes. The insertion of theTy1/Copia-like retrotransposon in thePH13H3gene attenuates the interaction between PH13 and GmCOP1s and increases the abundance of STFs protein, resulting in a stocky architecture in the natural population. The soybean accessions harboringPH13H3were selected during improvement and utilized by modern breeders at high latitude. Thephddouble mutants (harbors mutation in bothPH13andPHP) display excellent shade traits under high-density planting conditions, which can be further utilized to improve the yield at high latitudes. The YFP protein co-expressed with PH13 H1- Flag was used as a negative control. Following infiltration, the N. benthamiana plants were incubated at 25 °C for 12 h in the dark and then transferred to light growth conditions for an additional 36 h before IP analysis. The samples were harvested, ground, and treated with lysis buffer containing 1 mM MgCl 2 , 10 mM EDTA [pH 8.0], 1 mM PMSF, and 5 mM DTT, and Roche protease inhibitor cocktail. After centrifugation, the supernatant was incubated with anti-GFP trap agarose (Chromotek, catalog number gta-20) overnight at 4 °C, and rinsed three times with lysis buffer. The samples were boiled in SDS-PAGE sample buffer then analyzed using immunoblotting with anti-GFP antibody (at a 1:2500 dilution) followed by anti-Flag antibody (at a 1:2500 dilution). Light regimes White light (WL), blue light (400–499 nm), red light (600–699 nm), and far-red light (700–750 nm) LED panels (HiPoint brand, 14005-11145, Made in TAIWAN) were used separately or in combination as indicated (Supplementary Fig. 24 ). Low blue light (LBL) was achieved by filtering WL through two layers of yellow filters (no. 101, Lee Filters, CA), while low red: far-red light (L R:FR) was achieved by supplementing WL with far-red light [21] . The height of the LED was adjusted to maintain the Photosynthetic Photon Flux Density (PPFD) at about 500 μmol m −2 s −1 . The quality and intensity of light were measured by placing a HiPoint HR−350 spectrometer on top of the leaves. Statistical analyses For phenotypic investigation, at least five individual plants per accession were analyzed. The exact numbers of individuals ( n ) varying depending on the experiment were presented in the figure legends. The expression analysis were conducted by pooling at least three individual plants per tissue sample and performing at least three RT-qPCR reactions (technical replicates) for three biological replicates. Multiple comparisons were performed using GraphPad Prism 8.0 software with a two-way ANOVA and a two-sided Tukey test. For comparisons between two groups, two-tailed Student’s t -tests were conducted in Microsoft Excel to obtain p -values. The figure legends provide details on the statistical tests utilized for each experiment. Primers and accession number All primers used in this study are listed in Supplementary Data 8 . Gene sequences are available at the Phytozome database ( https://phytozome-next.jgi.doe.gov/info/Gmax_Wm82_a2_v1 ): PH13 / Glyma . 13G276700 , PHP/Glyma . 12G224600 , GmCOP1a / Glyma . 02G267800 , GmCOP1b / Glyma . 14G049700 , STF1 / Glyma . 08G302500 , STF2 / Glyma . 18G117100 , GmCRY1a / Glyma . 04G101500 , GmCRY1b/Glyma . 06G103200 , GmCRY1c / Glyma . 14G174200 and GmCRY1d/Glyma . 13G089200 . Reporting summary Further information on research design is available in the Nature Portfolio Reporting Summary linked to this article.